BRCA1 is an essential regulator of heart function and survival following myocardial infarction The tumour suppressor BRCA1 is mutated in familial breast and ovarian cancer but its role in protecting other tissues from DNA damage has not been explored. Here we show a new role for BRCA1 as a gatekeeper of cardiac function and survival. In mice, loss of BRCA1 in cardiomyocytes results in adverse cardiac remodelling, poor ventricular function and higher mortality in response to ischaemic or genotoxic stress. Mechanistically, loss of cardiomyocyte BRCA1 results in impaired DNA double-strand break repair and activated p53-mediated pro-apoptotic signalling culminating in increased cardiomyocyte apoptosis, whereas deletion of the p53 gene rescues BRCA1 -deficient mice from cardiac failure. In human adult and fetal cardiac tissues, ischaemia induces double-strand breaks and upregulates BRCA1 expression. These data reveal BRCA1 as a novel and essential adaptive response molecule shielding cardiomyocytes from DNA damage, apoptosis and heart dysfunction. BRCA1 mutation carriers, in addition to risk of breast and ovarian cancer, may be at a previously unrecognized risk of cardiac failure. Germline mutations in the tumour suppressor gene BRCA1 are highly penetrant for the increased risk of breast and ovarian cancer syndromes [1] , [2] . BRCA1 is mutated in up to 50% of inherited breast cancers and individuals who carry a defective copy of the gene have a 50–85% cumulative lifetime risk of developing breast cancer and a 12–60% chance of developing ovarian cancer [3] . BRCA1 functions as a 'caretaker' of genome stability and exerts multiple effects on key cellular processes involved in DNA damage repair, transcriptional regulation, ubiquitination and cell-cycle control [4] , [5] . The BRCA1 gene is composed of 24 exons and full-length BRCA1 encodes a ∼ 220-kD protein [6] , [7] . Exon 11 of the BRCA1 gene is the largest exon spanning ∼ 60% of the entire BRCA1 gene [3] . The exon 11 encoded domain of BRCA1 interacts and also colocalizes with RAD51 at the sites of DNA double-strand breaks (DSBs) to activate RAD51-mediated homologous recombination repair of DSBs [3] , [8] . Notably, BRCA1-deficient cells exhibit a deficit in RAD51-mediated homologous recombination repair of DSBs and hypersensitivity to DNA-damaging agents [9] . Un-repaired DNA damage is a trigger for apoptosis, which is important not only in the development of cancer syndromes but also represents a common pathophysiological basis for diverse chronic diseases including cardiovascular disease [10] , [11] , [12] , [13] . Indeed, ischaemia-induced DSBs [14] and apoptosis have been proposed as a key mechanism of cell death that occurs during cardiac ischaemia [15] , [16] , [17] . Apoptosis is also thought to contribute to the progressive loss of cardiac function with eventual transition towards overt cardiac failure, a leading cause of cardiac morbidity and death worldwide [15] , [16] , [17] . As BRCA1 has an integral role in promoting DNA damage repair, we hypothesized that BRCA1 regulates cardiomyocyte survival and that loss of function would provoke increased ischaemia-induced DNA damage, apoptosis and subsequent overt cardiac failure. We report herein for the first time that the loss of BRCA1 in cardiomyocytes leads to increased susceptibility to myocardial infarction (MI) and genotoxic drug (doxorubicin)-induced apoptosis and cardiac dysfunction. We also report that ischaemia leads to significantly higher DSBs and upregulation of BRCA1 expression, arguably to promote DSB repair in human adult and fetal ischaemic heart tissues. From a translational standpoint, these observations highlight a previously unrecognized role of BRCA1 as a gatekeeper of cardiac structure and function, and suggest that individuals carrying BRCA1 mutations may be at a previously unrecognized risk of cardiac failure, particularly in the setting of ischaemic or genotoxic stressors. Cardiomyocyte-specific BRCA1 knockout mice To delineate the role of BRCA1 in the heart, we first measured the basal transcript levels of BRCA1 in the different organs of wild-type (WT) mice and observed low expression of the BRCA1 transcript in murine hearts ( Fig. 1a ). In contrast, WT mice that had undergone a MI exhibited marked upregulation of BRCA1 in their remote myocardia, an effect that was significant within 36 h and that remained for a week post-MI ( Fig. 1b ). Next, to directly elucidate the involvement of BRCA1 in cardiac structure, function and survival, and to circumvent the embryonic lethality associated with systemic loss of BRCA1 (ref. 18 ), we applied the Cre-loxP system to specifically disrupt BRCA1 expression in cardiomyocytes. Conditional inactivation of BRCA1 in cardiomyocytes was achieved by crossing mice homozygous for the exon 11 floxed BRCA1 allele (BRCA1 fl/fl ) with hemizygous mice expressing Cre-recombinase under the control of the α -myosin heavy chain ( α MHC-Cre tg/ ) promoter as demonstrated in Fig. 1c [19] , [20] . Mice of the α MHC-Cre tg/ ;BRCA1 fl/fl background are denoted as cardiomyocyte-specific BRCA1 homozygous knockouts (CM-BRCA1 −/− ). Mice, regardless of their genotypes, were viable, fertile and were born in the expected Mendelian ratios. Analysis of genomic DNA from the heart, brain, liver and skeletal muscles revealed that the Cre -mediated recombined allele was only present in heart samples but not in the brain, liver and muscles of CM-BRCA1 +/− and CM-BRCA1 −/− mice ( Fig. 1d ). Successful deletion of BRCA1 at the protein level was confirmed by western blot analysis using an antibody that recognizes the exon 11 encoded C terminus of BRCA1. Graded cardiac BRCA1 protein levels were noted with the highest observed in samples from WT control mice, moderate in CM-BRCA1 +/− mice and the lowest in CM-BRCA1 −/− mice ( Fig. 1e , full blots are shown in Supplementary Figure S2 ). Although BRCA1 immunostaining of left ventricular (LV) sections further confirmed reduced BRCA1 expression in the cardiomyocytes of CM-BRCA1 +/− and CM-BRCA1 −/− mice, BRCA1 expression in most of the non-cardiomyocytes was found to be similar across the study groups ( Fig. 1f ). Taken together, these findings validate the successful generation of mice with cardiomyocyte-specific inactivation of full-length BRCA1. 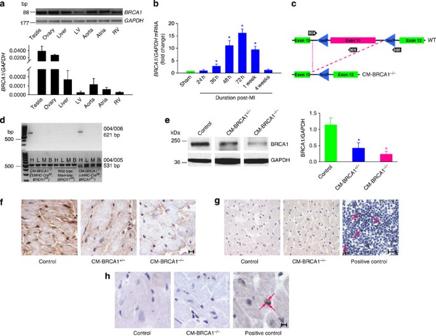Figure 1: BRCA1 expression in WT mice and characterization of CM-BRCA1−/−mice. (a) BRCA1 gene expression in tissues from WT mice. RV, right ventricle;n=3–4. (b) CardiacBRCA1transcript levels in WT mice post-MI;n=4, *P<0.01 versus sham-operated mice (pair-wise fixed reallocation randomization test). (c) Scheme ofCre-mediated deletion of exon 11 of theBRCA1gene. Black arrows denote binding sites of primers used for genotyping. (d) Genotypic identification of cardiomyocyte-specificBRCA1knockout mice. Genomic amplification of the 531 bp product of primer pair 004/005 indicates the presence of exon 11. Presence of the 621 bp product of primer pair 004/006 indicates the absence of the binding site for primer 005. CM-BRCA1+/−: αMHC-Cretg/;BRCA1fl/+mice; CM-BRCA1−/−: αMHC-Cretg/;BRCA1fl/flmice; H: heart; L: liver; M: skeletal muscles; B: brain. (e) Western blots of heart samples using an exon 11 splice variant-specific antibody of BRCA1. Protein bands shown are from non-adjacent lanes on the same gel.n=4–5, *P<0.01 versus control group (analysis of variance with post-hoc Bonferroni's correction). (f) Representative micrographs for baseline cardiac BRCA1 levels. Brown areas denote BRCA1 expression with haematoxylin counterstaining appearing blue. Scale bar, 20 μm. (g) Extent of apoptosis (TUNEL) in LV sections.n=3–4, scale bar, 50 μm. (h) DNA DSBs (γH2A.X foci formation) in LV sections. Liver and LV sections from doxorubicin-treated (10 mg kg−1, intraperitoneally 7 days before euthanasia) control mice were used for positive control assessments of γH2A.X and TUNEL staining, respectively.n=3–4, scale bar, 10 μm. Error bars inaandb, anderepresent s.e.m. and s.d,. respectively. Figure 1: BRCA1 expression in WT mice and characterization of CM-BRCA1 −/− mice. ( a ) BRCA1 gene expression in tissues from WT mice. RV, right ventricle; n =3–4. ( b ) Cardiac BRCA1 transcript levels in WT mice post-MI; n =4, * P <0.01 versus sham-operated mice (pair-wise fixed reallocation randomization test). ( c ) Scheme of Cre -mediated deletion of exon 11 of the BRCA1 gene. Black arrows denote binding sites of primers used for genotyping. ( d ) Genotypic identification of cardiomyocyte-specific BRCA1 knockout mice. Genomic amplification of the 531 bp product of primer pair 004/005 indicates the presence of exon 11. Presence of the 621 bp product of primer pair 004/006 indicates the absence of the binding site for primer 005. CM-BRCA1 +/− : α MHC-Cre tg/ ;BRCA1 fl/+ mice; CM-BRCA1 −/− : α MHC-Cre tg/ ;BRCA1 fl/fl mice; H: heart; L: liver; M: skeletal muscles; B: brain. ( e ) Western blots of heart samples using an exon 11 splice variant-specific antibody of BRCA1. Protein bands shown are from non-adjacent lanes on the same gel. n =4–5, * P <0.01 versus control group (analysis of variance with post-hoc Bonferroni's correction). ( f ) Representative micrographs for baseline cardiac BRCA1 levels. Brown areas denote BRCA1 expression with haematoxylin counterstaining appearing blue. Scale bar, 20 μm. ( g ) Extent of apoptosis (TUNEL) in LV sections. n =3–4, scale bar, 50 μm. ( h ) DNA DSBs (γH2A.X foci formation) in LV sections. Liver and LV sections from doxorubicin-treated (10 mg kg −1 , intraperitoneally 7 days before euthanasia) control mice were used for positive control assessments of γH2A.X and TUNEL staining, respectively. n =3–4, scale bar, 10 μm. Error bars in a and b , and e represent s.e.m. and s.d,. respectively. Full size image Cardiomyocyte BRCA1 loss and the unstressed heart The baseline (10–12 weeks old) cardiac structure and function of CM-BRCA1 −/− mice and their WT control littermates were indistinguishable ( Table 1 ). The WT control group included littermates with the BRCA1 +/+ , BRCA1 fl/+ , BRCA1 fl/fl and α MHC-Cre tg/ ;BRCA1 +/+ genotypes. Although high levels of Cre-recombinase in the heart have been associated with cardiomyopathy in aged mice, this pathology is evident only in mice that express Cre-recombinase 50 to 100 times greater than that in TG9, a α MHC-Cre -transgenic strain that does not develop congestive heart failure [21] . Nonetheless, to exclude the possible involvement of Cre -mediated cardiomyopathy in our model, parallel studies were conducted on littermates expressing the Cre -only (α MHC-Cre tg/ ;BRCA1 +/+ ) background. As our results indicated no differences between the Cre -only mice and the other WT control littermates at baseline and after MI, the former animals were included in the WT control group. Molecular work on apoptosis, as evaluated by TdT-mediated dUTP nick end labeling (TUNEL) staining of LV sections, indicated similar patterns between the groups ( Fig. 1g ). The extent of DSBs, as measured by γH2A.X foci formation ( Fig. 1h ), also did not reveal any baseline differences between hearts from CM-BRCA1 −/− mice and their WT control littermates. Hence, in the absence of stress, cardiomyocyte-specific deletion of BRCA1 resulted in no grossly apparent cardiac phenotype. Table 1 Echocardiographic assessments indicate that control and CM-BRCA1 −/− mice exhibit similar cardiac function at baseline. Full size table Cardiomyocyte BRCA1 loss and post-MI mortality To explore the function of BRCA1 in the heart, we monitored the survival of CM-BRCA1 −/− mice, CM-BRCA1 +/− mice and their WT control littermates for 22 weeks following MI. Post-MI mortality in CM-BRCA1 −/− mice was profoundly higher relative to that for their WT control littermates and CM-BRCA1 +/− mice demonstrated intermediate but significantly higher post-MI mortality compared with the WT controls ( Fig. 2a ). Tachypnea, hunched back posture and raised fur were the most evident visual symptoms before death in CM-BRCA1 −/− mice in comparison with the WT control littermates. At post-MI autopsies, pleural effusion and pulmonary oedema were consistently observed in CM-BRCA1 −/− mice but not in the control mice. To determine if the elevated post-MI mortality observed with CM-BRCA1 −/− mice is associated with larger infarct sizes, myocardial infarcts 4 weeks post-MI were measured and indeed, as shown in Fig. 2b , CM-BRCA1 −/− mice exhibited a larger mean infarct size relative to their WT control littermates. There were no differences in the areas at risk between the groups 24 h post-MI ( Fig. 2c ). Furthermore, a ∼ 1.5-fold increase in the LV radius to LV wall thickness (r/h) ratio was observed in CM-BRCA1 −/− mice relative to the WT control littermates ( Fig. 2d ). Collectively, these findings demonstrate that loss of BRCA1 in cardiomyocytes is associated with poor cardiac outcomes, adverse cardiac remodelling and increased mortality in response to ischaemic stress. 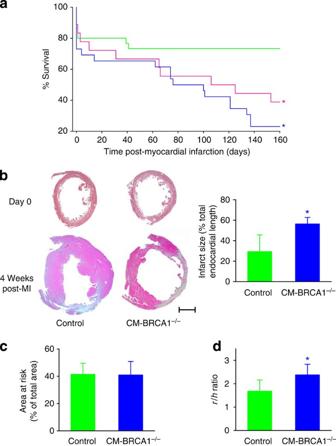Figure 2: Loss of cardiomyocyte-specific BRCA1 leads to increased mortality following myocardial infarction. (a) Post-MI Kaplan–Meier survival curves for WT control (green;n=30), CM-BRCA1+/−(magenta;n=18) and CM-BRCA1−/−(blue;n=26) littermates. *P<0.01 (Log-rank and Gehan–Wilcoxon tests). (b) Representative baseline and post-MI (4 weeks) myocardial sections (scale bar, 1 mm). Macroscopic measurements of infarct sizes.n=9–11. (c) Quantification of post-MI (24 h) myocardial areas at risk;n=3–4. (d) Post-MI LV radius-to-septum thickness ratio (r/h);n=10. Error bars inb–drepresent s.d. with *P<0.05 versus control values in all cases (Student'st-test). Figure 2: Loss of cardiomyocyte-specific BRCA1 leads to increased mortality following myocardial infarction. ( a ) Post-MI Kaplan–Meier survival curves for WT control (green; n =30), CM-BRCA1 +/− (magenta; n =18) and CM-BRCA1 −/− (blue; n =26) littermates. * P <0.01 (Log-rank and Gehan–Wilcoxon tests). ( b ) Representative baseline and post-MI (4 weeks) myocardial sections (scale bar, 1 mm). Macroscopic measurements of infarct sizes. n =9–11. ( c ) Quantification of post-MI (24 h) myocardial areas at risk; n =3–4. ( d ) Post-MI LV radius-to-septum thickness ratio (r/h); n =10. Error bars in b – d represent s.d. with * P <0.05 versus control values in all cases (Student's t -test). Full size image Cardiomyocyte BRCA1 loss and post-MI cardiac changes Echocardiographic assessment of cardiac structure and function post-MI revealed reduced ejection fraction and fractional shortening ( Fig. 3a ) as well as increased ventricular dimensions in CM-BRCA1 −/− mice compared with their WT control littermates ( Fig. 3b ). Congruent with these observations, invasive pressure–volume measurements also indicated twofold greater end-systolic and end-diastolic volumes and 50% lower ejection fractions in CM-BRCA1 −/− mice post-MI ( Table 2 ; Fig. 3c ). The reduced first derivative of pressure during isovolumic contraction ( dP/dt max) and relaxation ( dP/dt min) along with the rightward shift of the volume intercept ( Fig. 3d,e ) suggest that the impairment in cardiac function in CM-BRCA1 −/− mice arose to a large degree because of the exaggerated LV dilation post-MI. CM-BRCA1 −/− mice displayed a decrease in heart weight/body weight ratio (5.3±0.9 and 4.1±0.3; WT versus CM-BRCA1 −/− , P <0.01; Student's t -test) in response to MI, when compared with their WT control littermates. We also analysed the transcript levels of brain natriuretic peptide, which is an established marker for the heart failure and demonstrate a significant upregulation in the hearts of CM-BRCA1 −/− in comparison to the WT control littermates post-MI ( Fig. 3f ). 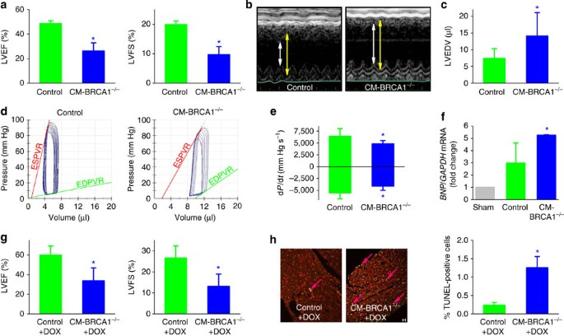Figure 3: Loss of cardiomyocyte-specific BRCA1 leads to aberrant cardiac changes following ischaemic and genotoxic stress. (a) LV performance (ejection fraction (LVEF) and fractional shortening (LVFS)) 4 weeks post-MI, as assessed by echocardiography;n=4–6. (b) Representative M-mode echocardiograms with LV end systolic and end diastolic diameters annotated in white and yellow, respectively. (c) LV end diastolic volume (LVEDV).n=9–11. (d) Representative pressure–volume loops of infarcted hearts (4 weeks post-MI) from CM-BRCA1−/−mice and their WT control littermates. (e)dP/dtvalues.n=9–11. (f)BNPexpression 4 weeks post-MI as determined by real-time PCR on cDNA synthesized from total LV RNA.GAPDHwas used as an endogenous control.n=5–6. (g) Echocardiography results showing LV function. (h) Cardiomyocyte apoptosis (TUNEL staining; arrows) 7 days following a single treatment with 10 mg kg−1(intraperitoneal) doxorubicin. Scale bar, 10 μm,n=4–6. Error bars in (a,c,e–h) represent s.d. with *P<0.05 versus control values in all cases (Student'st-test). Figure 3: Loss of cardiomyocyte-specific BRCA1 leads to aberrant cardiac changes following ischaemic and genotoxic stress. ( a ) LV performance (ejection fraction (LVEF) and fractional shortening (LVFS)) 4 weeks post-MI, as assessed by echocardiography; n =4–6. ( b ) Representative M-mode echocardiograms with LV end systolic and end diastolic diameters annotated in white and yellow, respectively. ( c ) LV end diastolic volume (LVEDV). n =9–11. ( d ) Representative pressure–volume loops of infarcted hearts (4 weeks post-MI) from CM-BRCA1 −/− mice and their WT control littermates. ( e ) dP/dt values. n =9–11. ( f ) BNP expression 4 weeks post-MI as determined by real-time PCR on cDNA synthesized from total LV RNA. GAPDH was used as an endogenous control. n =5–6. ( g ) Echocardiography results showing LV function. ( h ) Cardiomyocyte apoptosis (TUNEL staining; arrows) 7 days following a single treatment with 10 mg kg −1 (intraperitoneal) doxorubicin. Scale bar, 10 μm, n =4–6. Error bars in ( a , c , e – h ) represent s.d. with * P <0.05 versus control values in all cases (Student's t -test). Full size image Table 2 Echocardiographic post-MI invasive pressure-volume assessments. Full size table To confirm the robustness of our observations, we evaluated the cardiac phenotype of CM-BRCA1 −/− mice that had been subjected to an alternative stressor, the chemotherapeutic agent doxorubicin (single dose, 10 mg kg −1 , intraperitoneally). We report that CM-BRCA1 −/− mice treated with doxorubicin exhibit worse cardiac function and more cardiomyocyte apoptosis compared with control mice 7-days post-treatment ( Fig. 3g,h ). Taken together, these data indicate that deficiency of full-length BRCA1 in cardiomyocytes results in increased susceptibility to cardiac failure under both ischaemic and genotoxic conditions. Cardiomyocyte BRCA1 loss and cardiomyocyte death post-MI Programmed cardiomyocyte death has been suggested to underlie progressive ventricular remodelling and ischaemic cardiac failure [16] , [22] . As BRCA1 exerts a multitude of effects to promote DNA repair and limit apoptotic cell death pathways, we postulated that cardiomyocyte specific loss of BRCA1 may provoke cardiac failure through a similar mechanism. We demonstrate that the prevalence of apoptotic cardiomyocyte nuclei, as identified by TUNEL staining, was higher in LV sections from CM-BRCA1 +/− and CM-BRCA1 −/− mice compared with those from their WT control littermates post-MI ( Fig. 4a ). To discriminate apoptosis in cardiomyocytes from non-myocytes, myocardial sections were doubly stained for TUNEL and the cardiomyocyte-specific structural protein α-myosin heavy chain. This data was further confirmed by immunostaining for caspase-3 and western blot for cleaved caspase-3, which was increased post-MI in the LV sections of CM-BRCA1 −/− in comparison with WT control littermates ( Fig. 4b,c ). 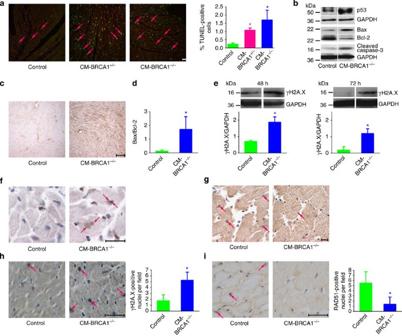Figure 4: Cardiomyocyte-specificBRCA1loss increases MI-induced pro-apoptotic cardiac events and impairs repair of MI-induced DNA DSBs. (a) TUNEL-positive nuclei (arrows) in LV sections 4 weeks post-MI. Magnification ×200. Scale bar 10 μm,n=4–5. (b) Western blots for p53, Bax, Bcl-2, and cleaved caspase-3. (c) Total caspase-3 immunostaining (brown). Scale bar 100 μm. (d) Bax/Bcl-2 ratios in the remote myocardium 4 weeks post-MI.n=4–5. (e) Western blots for γH2A.X levels in hearts harvested 48 and 72 h post-MI. Forbande, protein bands shown are from non-adjacent lanes on the same gel. (f) Immunohistochemical staining showing γH2A.X foci (arrows) in LV sections obtained 72 h post-MI. Scale bar 10 μm.n=4–5. (g) RAD51 foci formation (arrows) in LV sections harvested 72 h post-MI. Magnification ×60. Scale bar 100 μm. Staining (arrows) and quantification of (h) γH2A.X and (i) RAD51-foci in LV sections from doxorubicin-treated mice. Magnification ×100. Scale bar 10 μm,n=6. Error bars ina,d,e,h,irepresent s.d. with *P<0.05 versus control group in all cases (Student'st-test). Figure 4: Cardiomyocyte-specific BRCA1 loss increases MI-induced pro-apoptotic cardiac events and impairs repair of MI-induced DNA DSBs. ( a ) TUNEL-positive nuclei (arrows) in LV sections 4 weeks post-MI. Magnification ×200. Scale bar 10 μm, n =4–5. ( b ) Western blots for p53, Bax, Bcl-2, and cleaved caspase-3. ( c ) Total caspase-3 immunostaining (brown). Scale bar 100 μm. ( d ) Bax/Bcl-2 ratios in the remote myocardium 4 weeks post-MI. n =4–5. ( e ) Western blots for γH2A.X levels in hearts harvested 48 and 72 h post-MI. For b and e , protein bands shown are from non-adjacent lanes on the same gel. ( f ) Immunohistochemical staining showing γH2A.X foci (arrows) in LV sections obtained 72 h post-MI. Scale bar 10 μm. n =4–5. ( g ) RAD51 foci formation (arrows) in LV sections harvested 72 h post-MI. Magnification ×60. Scale bar 100 μm. Staining (arrows) and quantification of ( h ) γH2A.X and ( i ) RAD51-foci in LV sections from doxorubicin-treated mice. Magnification ×100. Scale bar 10 μm, n= 6. Error bars in a , d , e , h , i represent s.d. with * P <0.05 versus control group in all cases (Student's t -test). Full size image BRCA1-null mutants die embryonically due to p53 hyperactivity but this embryonic lethality can be partially rescued by p53 deficiency [18] . Upregulation of p53 due to hypoxia or forced expression of p53 is sufficient to induce apoptosis in cardiomyocytes [23] , and importantly, p53-null mice subjected to MI exhibit reduced apoptosis and improved survival [24] . In line with these findings, we also demonstrate an increase in total p53 expression in the hearts of CM-BRCA1 −/− compared with their WT control littermates post-MI ( Fig. 4b ). The p53-dependent apoptotic signalling pathway involves the Bcl-2 family of proteins (Bcl-2 and Bax), which are recognized as major regulators of cardiomyocyte apoptosis and have been implicated as a critical mediator of cardiomyocyte survival decisions during heart failure [16] , [25] , [26] . Indeed, the increase in cardiomyocyte apoptosis in CM-BRCA1 −/− mice was associated with a loss of myocardial pro-survival Bcl-2 with a concomitant increase in pro-apoptotic Bax leading to a ∼ 12.5 fold increase in the Bax to Bcl-2 ratio ( Fig. 4b,d ), hence shifting the balance from a survival to apoptotic milieu. This shift was further associated with elevated levels of total and cleaved caspase-3 compared with the corresponding control group ( Fig. 4b , full blots are shown in Supplementary Figure S3 ). Cardiomyocyte BRCA1 loss and DSB repair post-MI Given the central role of BRCA1 in DNA DSB repair, we postulated that an ischaemic insult in the setting of BRCA1 deficiency may result in an increased burden of DSBs, setting the stage for progressive cardiomyocyte apoptosis [4] , [5] , [27] . One of the first steps in the cellular response to DSBs is phosphorylation of histone H2A.X at Ser139, referred to as γH2A.X [4] , [28] . At these sites of DNA damage, γH2A.X appears to have a critical function in the recruitment of additional DNA repair factors and represents an early and sensitive marker of chromatin modification before cells undergo the process of repair or apoptosis [28] . Indeed, a ∼ 2.5-fold higher expression of γH2A.X was observed in cardiomyocyte nuclei from the hearts of CM-BRCA1 −/− mice compared with corresponding sections from control animals 48 h post-MI ( Fig. 4e , full blots are shown in Supplementary Figure S3 ). Although after 72 h, this DNA damage signal resolved in control mice, and a persistent γH2A.X signal was observed in LV sections of CM-BRCA1 −/− mice ( Fig. 4e,f ). Moreover, BRCA1 is required for RAD51-foci formation at the sites of DNA damage, which then activates RAD51-mediated repair of DSBs [29] . Therefore, it became of interest to evaluate RAD51-foci formation in myocardial samples from control and CM-BRCA1 −/− mice. Although control mice exhibited evidence for post-MI RAD51-foci formation, such foci were significantly reduced in number in mice with cardiomyocyte-specific loss of BRCA1 ( Fig. 4g ). Increased doxorubicin-induced cardiac dysfunction and apoptosis observed in CM-BRCA1 −/− mice correlated with increased levels of DSBs in the left ventricle in comparison with the WT control littermates ( Fig. 4h ). Degree of DSBs repair was measured by the extent of RAD51-foci formation, which demonstrated significantly reduced RAD51-foci in the left ventricle of doxorubicin-treated CM-BRCA1 −/− mice ( Fig. 4i ). Collectively, these data suggest that a reduction in cardiomyocyte BRCA1 activity leads to unresolved DNA damage and the absence of effective homologous recombination repair sets the stage for increased p53-mediated apoptosis and ensuing cardiac failure. Heterozygous p53 loss rescues BRCA1-deficient mice from MI As previously stated, the phenotype associated with systemic loss of BRCA1 is attenuated with concomitant loss of p53 (ref. 18 ). Hence it became plausible to explore the effect of BRCA1 loss in cardiomyocyte with compound systemic deletion of p53 in the setting of ischaemic stress. To establish the role for p53 activation in the impaired cardiac stress response observed in BRCA1-deficient mice, we crossed α MHC-Cre tg/ ;BRCA1 fl/fl mice with p53 +/− mutants to generate mice that have one allele of BRCA1 in their cardiomyocytes along with the systemic loss of one allele of p53 ( α MHC-Cre tg/ ;BRCA1 fl/+ ;p53 +/− otherwise denoted as CM-BRCA1 +/− ;p53 +/− ). We report that CM-BRCA1 +/− ;p53 +/− mice are protected against MI-induced apoptosis and cardiac dysfunction in comparison to CM-BRCA1 +/− mice ( Fig. 5a,b ). 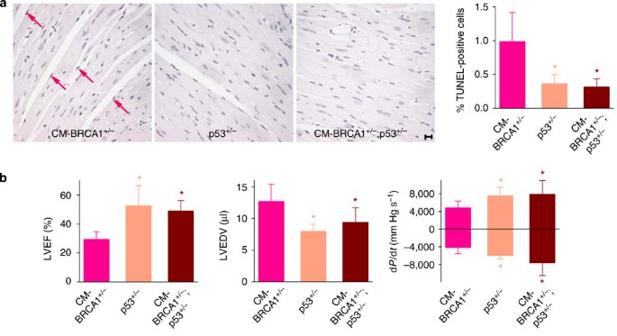Figure 5: Deletion of a singlep53allele reverses the cardiac dysfunction associated with cardiomyocyte-specificBRCA1loss. (a) TUNEL-positive nuclei (arrows) in the post-MI remote myocardium. Magnification ×40. Scale bar 10 μm,n=5–7. (b) Echocardiography results showing LV function as per LV ejection fraction, (LVEDV) anddP/dtvalues.n=6–8. Error bars represent s.d. with *P<0.05 versus CM-BRCA1+/−group in all cases (analysis of variance with post-hoc Bonferroni's corrections). Figure 5: Deletion of a single p53 allele reverses the cardiac dysfunction associated with cardiomyocyte-specific BRCA1 loss. ( a ) TUNEL-positive nuclei (arrows) in the post-MI remote myocardium. Magnification ×40. Scale bar 10 μm, n =5–7. ( b ) Echocardiography results showing LV function as per LV ejection fraction, (LVEDV) and dP/dt values. n =6–8. Error bars represent s.d. with * P <0.05 versus CM-BRCA1 +/− group in all cases (analysis of variance with post-hoc Bonferroni's corrections). Full size image To further support these findings and also to mimic clinically relevant human BRCA1-defficient conditions, we generated mice with a compound systemic deletion of one allele of both BRCA1 and p53 . Following MI, compound heterozygous BRCA1 +/Δ11 ;p53 +/− mice demonstrated that systemic loss of one allele of p53 rescued BRCA1 +/Δ11 heterozygous mice against MI-induced cardiac dysfunction (ejection fraction: 34.0±4% and 48.9±4.9% for BRCA1 +/Δ11 and BRCA1 +/Δ11 ;p53 +/− , respectively; P <0.01; Student's t -test). Thus, loss of BRCA1 provokes ischaemia-induced cardiomyocyte apoptosis through upregulation of p53-mediated cell death pathways, which is causally implicated in ischaemic heart failure. Cardiac BRCA1 is upregulated following ischaemia in humans To further explore the clinical relevance of BRCA1, we assessed BRCA1 expression in human cardiac samples following ischaemic stress. First, we utilized a well-validated model of human atrial cardiac ischaemia and reperfusion [30] wherein atrial biopsies were obtained intraoperatively from patients before and after initiation of cardiopulmonary bypass (CPB). We measured BRCA1 expression levels and the extent of DSBs by immunoblot and immunostaining. BRCA1-mediated DSB repair was evaluated by immunostaining for RAD51. We report that human atria subjected to perioperative ischaemia and reperfusion (post-cardioplegia (CP)/CPB) demonstrated higher BRCA1 expression ( Fig. 6a,b ). Increased BRCA1 in the post-CP/CPB atrial biopsies were associated with significantly higher levels of γH2A.X expression and γH2A.X-foci formation demonstrating more ischaemia-induced DSBs ( Fig. 6c,d ). This phenotype was accompanied with higher extent of BRCA1-mediated DSB-repair as evident by increased numbers of RAD51-foci compared with those from pre-CPB subjects ( Fig. 6d ). 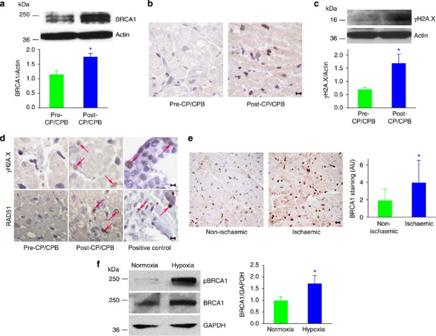Figure 6: BRCA1 protein levels are elevated in human adult cardiac tissues and fetal cardiomyocytes following exposure to ischaemic conditions. Atrial appendages were obtained pre- and post-CPB from patients undergoing coronary artery bypass graft surgery. Atrial biopsies were sectioned and total proteins were isolated to perform western blotting and immunohistochemical staining. (a) Representative immunoblots and immunoband quantification for atrial appendage BRCA1 and actin expressions.n=4, *P<0.05 versus pre-CP/CPB group. (b) Representative photomicrograph for BRCA1 expression (brown) in human atrial appendages. Scale bar 10 μm,n=4–5. (c) Representative immunoblots and immunoband quantification for γH2A.X and actin. Scale bar 10 μm,n=4–11, *P<0.05 versus pre-CP/CPB group. (d) Representative photomicrograph for γH2A.X and RAD51 staining of human atrial sections. Human placenta sections were used as a positive control. Scale bar 10 μm,n=4–5. (e) BRCA1 immunostaining (brown) in adult human LV myocardial sections. Scale bar 10 μm,n=4, *P<0.05 versus non-ischaemic group. (f) Representative immunoblots and immunoband quantification for BRCA1, phospho-BRCA1 and GAPDH in primary human fetal cardiomyocyte cultures following exposure to 48 h of hypoxic conditions.n=3, *P<0.05 versus normoxic group (Student'st-test). Figure 6: BRCA1 protein levels are elevated in human adult cardiac tissues and fetal cardiomyocytes following exposure to ischaemic conditions. Atrial appendages were obtained pre- and post-CPB from patients undergoing coronary artery bypass graft surgery. Atrial biopsies were sectioned and total proteins were isolated to perform western blotting and immunohistochemical staining. ( a ) Representative immunoblots and immunoband quantification for atrial appendage BRCA1 and actin expressions. n =4, * P <0.05 versus pre-CP/CPB group. ( b ) Representative photomicrograph for BRCA1 expression (brown) in human atrial appendages. Scale bar 10 μm, n =4–5. ( c ) Representative immunoblots and immunoband quantification for γH2A.X and actin. Scale bar 10 μm, n =4–11, * P <0.05 versus pre-CP/CPB group. ( d ) Representative photomicrograph for γH2A.X and RAD51 staining of human atrial sections. Human placenta sections were used as a positive control. Scale bar 10 μm, n =4–5. ( e ) BRCA1 immunostaining (brown) in adult human LV myocardial sections. Scale bar 10 μm, n =4, * P <0.05 versus non-ischaemic group. ( f ) Representative immunoblots and immunoband quantification for BRCA1, phospho-BRCA1 and GAPDH in primary human fetal cardiomyocyte cultures following exposure to 48 h of hypoxic conditions. n =3, * P <0.05 versus normoxic group (Student's t -test). Full size image Second, to extend our observations to a model of chronic ischaemic heart disease, we obtained ventricular biopsies from patients undergoing open-heart surgery. BRCA1 protein levels in ventricular biopsies from patients undergoing valvular surgery without clinical signs and symptoms of ischaemia (non-ischaemic group) were compared with tissues from patients with documented coronary artery disease undergoing coronary artery bypass surgery (ischaemic group). We report that human ventricular tissues from patients with ischaemic heart disease demonstrated higher levels of BRCA1 compared with those from subjects without ischaemic heart disease ( Fig. 6e ). Third, to evaluate whether this ischaemia-induced upregulation of BRCA1 is specific to cardiomyocytes, and is not dependent on non-myocyte factors, we cultured primary human fetal cardiomyocytes derived from normal hearts after elective pregnancy termination (gestational age 15–20 weeks) under normoxic and hypoxic environment [31] . We report a significant upregulation of total and phosphorylated BRCA1 in human fetal cardiomyocytes in response to hypoxia ( Fig. 6f ). The BRCA1 gene is classified as a 'tumour suppressor' and 'caretaker' on the basis of its proposed genome integrity maintenance functions [32] . Germ-line mutations in BRCA1 predominantly predispose carriers to breast and ovarian cancer in addition to other cancer syndromes [33] . BRCA1 is important for various cellular functions and exerts its effects on key cellular processes involved in DNA nucleotide excision and DSB repair, transcriptional regulation, ubiquitination and cell-cycle control [4] , [5] , [27] , [34] . Mice harbouring complete ablation of BRCA1 die embryonically and display neuroepithelial, proliferative and morphogenetic abnormalities [35] , [36] , [37] . The BRCA1 gene is composed of 24 exons. Exon 11 is the largest exon and covers ∼ 60% of the entire BRCA1 gene [3] . The exon 11 encoded domain interacts and colocalizes with RAD51 at the sites of DNA damage to activate RAD51-mediated repair of DSBs [3] , [8] . Mice with systemic deletion of exon 11 in the BRCA1 gene show recessive embryonic lethality due to impaired DNA damage-induced activation of BRCA1, compromised RAD51-dependent repair pathway and increased apoptosis [38] , [39] . To understand the DNA damage repair function of BRCA1 in mature cardiac muscles, we utilized the Cre-loxP system to delete exon 11 of the BRCA1 gene specifically in cardiomyocytes and successfully generated CM-BRCA1 −/− mice. Although the transcription and translation of the BRCA1 Δ11 splice variant cannot be ruled out, it should be noted that if translated, it would still not encode the major part of the C-terminus domain and therefore would be non-functional with respect to the DNA damage repair properties of BRCA1. Baseline cardiac morphology as well as indices of cardiac functions along with apoptosis and DNA damage were indistinguishable between CM-BRCA1 −/− and the WT control littermates. Strikingly, whereas almost 95% of the CM-BRCA1 −/− mice and ∼ 60% of the CM-BRCA1 +/− mice were dead at the end of the study period (22 weeks), corresponding mortality in the WT mice was only ∼ 20%. These mice died more frequently due to congestive heart failure and showed dilatation of the left ventricle. A closer analysis of the cardiac phenotype at 4 weeks post-MI revealed that CM-BRCA1 −/− mice had increased infarct sizes, poor cardiac function, reduced contractility, dilated left ventricles and blunted compensatory hypertrophy compared with WT mice. Ischaemia and accompanying hypoxic stress manifested with increased DNA breaks are the primary triggers for the induction of pro-apoptotic cascades leading to apoptotic cell death [40] , [41] . Given the central role of BRCA1 in DSB repair, we postulated that an ischaemic insult may result in an increased burden of DSBs and that under conditions of BRCA1 deficiency there may be accumulation of unresolved DSBs thereby setting the stage for cardiomyocyte apoptosis and cardiac dysfunction [4] , [5] , [27] . Congruent with our hypothesis, we observed ∼ 2.5 fold greater DSBs in hearts from CM-BRCA1 −/− mice compared with those from the control littermates 48 h post-MI. Cardiac DSBs were resolved 72 h post-MI in WT control littermates but were persistently present in the hearts of CM-BRCA1 −/− mice. Peak cardiac BRCA1 expression in WT mice occurred 72 h post-MI providing a clear indication that BRCA1 is required for repairing ischaemia-induced DSBs. This finding is further strengthened by the degree of RAD51-foci formation, another marker of DSB repair, which temporally correlated with MI-induced BRCA1 expression in WT littermates. The observation that the extent of RAD51-foci formation was reduced in the hearts of CM-BRCA1 −/− mice post-MI suggests accumulation of unresolved DSBs, which would accordingly shift the balance towards cardiomyocyte death. Ischaemia-induced increased mortality and cardiac dysfunction were further associated with significantly higher numbers of TUNEL-positive nuclei and cleaved caspase-3 expression demonstrating increased cardiomyocyte death in the hearts of CM-BRCA1 −/− mice compared with corresponding WT control littermates post-MI. Systemic loss of BRCA1-associated embryonic lethality in mice can be partially rescued by the heterozygous deletion of the tumour suppressor gene p53 [18] . Intriguingly, loss of p53 protects the heart from rupture and associated death, whereas overexpression of p53 induces cardiomyocyte apoptosis [24] , [42] , [43] , [44] . Therefore, we sought to determine if p53 is a modulator of cardiomyocyte apoptosis post-MI in CM-BRCA1 −/− mice. We found significantly higher p53 protein levels along with increased p53-regulated pro-apoptotic downstream target Bax post-MI in the hearts of CM-BRCA1 −/− mice. The most important factor in the p53-dependent survival and/or apoptotic signalling pathway is the shift in the ratio between the pro-apoptotic Bax and pro-survival molecule Bcl-2 (ref. 45 ), both of which are recognized as major regulators of cardiomyocyte apoptosis and/or survival decisions during heart failure [25] , [26] . We observed that the MI-induced increase in cardiomyocyte apoptosis in CM-BRCA1 −/− mice was associated with an ∼ 10 fold increase in the Bax to Bcl-2 ratio, shifting the balance from a survival to an apoptotic milieu. As the systemic loss of BRCA1-associated embryonic lethality in mice can be partially rescued by the heterozygous deletion of p53 (refs 18 , 46 ), we investigated how deletion of one allele of p53 would affect the MI-induced cardiac phenotype associated with cardiomyocyte-specific loss of BRCA1. To this aim, we generated double heterozygous knockout mice (CM-BRCA1 +/− ; p53 +/− ). We report that the post-MI phenotype associated with loss of full-length BRCA1 could be prevented with systemic deletion of one allele of p53 , such that the heart from the these mice show reduced apoptosis as well as improved cardiac function and contractility post-MI. We further confirm the direct role of p53 in BRCA1 deficiency-associated post-MI cardiac phenotype by systemically deleting one allele of both BRCA1 and p53 , which mimics more of a human BRCA1-haploinsufficient condition and demonstrate that deletion of one allele of p53 was able to rescue the BRCA1-deficiency-associated MI-induced cardiac phenotype. Chemotherapeutic agents function by directly or indirectly damaging DNA through various mechanisms [47] . Doxorubicin is a potent chemotherapeutic agent used for a wide variety of malignancies, but the clinical utility has been limited by its dose-dependent cardiotoxicity, which eventually results in refractory cardiac dysfunction [48] . Doxorubicin induces DSBs [49] and BRCA1 has been previously implicated in the repair of DSBs [4] . Thus the role of BRCA1 in response to doxorubicin-induced cardiotoxicity is an important subject for investigation. In our hands, CM-BRCA1 −/− mice showed reduced cardiac performance, increased DSBs, reduced DSB repair and enhanced cardiomyocyte death in comparison to the WT mice following treatment with doxorubcin. Of note, we provide herein evidence of clinical relevance to our in vivo observations. We report that ischaemia significantly upregulated BRCA1 expression in adult human atrial and ventricular tissues, and also in human fetal cardiomyocytes. Importantly, we also show that ischaemia significantly induced DSBs in human atrial tissues. BRCA1 physically interacts with RAD51 to regulate RAD51 nuclear transport, which is required for DSB repair [29] . We propose that ischaemia induced-BRCA1 upregulation is associated with increased DSB repair and this is confirmed by greater RAD51-foci formation in ischaemic atrial tissues. We demonstrate for the first time that BRCA1 protects atrial and ventricular tissues against DSBs by promoting DSB repair through RAD51 interaction, and thus loss of function or BRCA1 haplo-insufficiency may lead to impaired DSB repair with subsequent accumulation of DNA damage, apoptosis and/or cardiac dysfunction. Taken together this study provides evidence that in the heart BRCA1 mediates a survival pathway that acts to block the onset of apoptosis resulting in cardiac dysfunction following ischaemic or genotoxic stress. Our data identifying BRCA1 as an essential and novel regulator of heart function affords important translational implications. From a therapeutic standpoint, our data suggest that BRCA1 may represent a novel therapeutic target to limit cardiac failure, a leading cause of death worldwide [50] . From an epidemiological standpoint, these observations provide important clues regarding a potential susceptibility of BRCA1 mutation carriers to cardiovascular disease, in addition to the well-documented predisposition towards cancer syndromes. Recent data suggest that BRCA1/2 mutation carriers exhibit an increase in non-neoplastic death particularly at older ages [51] , [52] . Although the causes of non-neoplastic death in the reported population remain unknown, our data raise the possibility that the excess mortality may be due to increased rates of death from ischaemic heart disease. Finally, from a pharmacogenomic point of view, this data may indicate a heightened susceptibility of BRCA1 mutation carriers to anthracycline-induced cardiac failure [53] , a cornerstone of chemotherapy for breast and ovarian cancer. Animal studies All animal procedures were performed in accordance with the guidelines of the Canadian Council on Animal Care and were approved by the St Michael's Animal Care Committee. Studies were performed on 10–12 weeks old male mice housed in a climate-controlled (temperature 22–24 °C, humidity 40–60%) light-regulated room with a 12 h light:12 h dark cycle. Each cage accommodated up to five mice and was ventilated at 60 ACH. Mice were maintained on irradiated Teklad Global 18% Protein Rodent Diet pellets (Harlan Laboratories) and had ad libitum access to reverse osmosis water throughout the acclimatization and study windows. C57Bl/6J mice were obtained from the Jackson Laboratory. CM-BRCA1 −/− mice were generated using the Cre-loxP technology on a mixed background. Briefly, as shown in Supplementary Figure S1 and Fig. 1c , mice homozygous for the exon 11 floxed BRCA1 allele (BRCA1 fl/fl ; NCI, MHCC, Mouse Repository; strain# 01XC8, strain name: Brca1 tm2Cxd ) [3] were crossed with hemizygous mice expressing Cre-recombinase under the control of the α -myosin heavy chain (αMHC- Cre tg/ ) promoter [19] . Mice of the αMHC- Cre tg/ ;BRCA1 fl/+ combination were denoted as cardiomyocyte-specific BRCA1 heterozygous (CM-BRCA1 +/− ) and those with the αMHC- Cre tg/ ;BRCA1 fl/fl combination as cardiomyocyte-specific BRCA1 homozygous (CM-BRCA1 −/− ) knockouts. Mice were genotyped using routine PCR with the following sets of primers: 004:5′-CTGGGTAGTTTGTAAGCATGC-3′ 005:5′-CAATAAACTGCTGGTTCTAGG-3′ 006:5′-CTGCGAGCAGTCTTCAGAAAG-3′ αMHC- Cre transgene Forward-5′-ATGACAGACAGATCCCTCCTATCTCC-3′ Reverse-5′-CTCATCACTCGTTGCATCGAC-3′ To generate CM-BRCA1 −/− mice with a p53 +/− background, αMHC- Cre tg/ ;BRCA1 fl/fl mice were crossed with p53 +/− mice (Jackson Laboratory; stock# 002101, strain name: B6.129S2-Trp53 tm1Tyj/J ). This resulted in mice with one allele of BRCA1 in their cardiomyocytes while presenting with systemic loss of one allele of p53 (αMHC Cre tg/ ;BRCA1 fl/+ ;p53 +/− denoted as CM-BRCA1 +/− ;p53 +/− ). B6.129S2-Trp53 tm1Tyj/J mice were genotyped as suggested by Jackson Laboratory. We also utilized BRCA1 +/Δ11 mice with a p53 +/− background by crossings BRCA1 +/Δ11 mice with p53 +/− mice [54] . Experimental MI Mice (10–12 weeks) underwent coronary artery ligation to induce MI as previously published [55] , [56] , [57] , [58] . Analgesia was provided with 0.1 mg kg −1 Buprenex before deep anaesthesia was induced with isoflurane in an anaesthetic chamber. The surgical plane was maintained under 1–1.5% isoflurane. Mice were intubated with a 20-G intravenous cannula that was subsequently connected to a mouse ventilator (Minivent, Harvard Apparatus) via a Y-shaped connector. Mechanical ventilation was accomplished with 100% oxygen at a tidal volume of 200 μl and a respiratory rate of 133 cycles per min. The site above the left 4th intercostal space was disinfected before an incision ( ∼ 1 cm in length) perpendicular to the sternum was made. The ribs were retracted with 4-0 silk suture and the pericardium pulled apart gently to render a clear view of the heart and its vascular structures. The left coronary artery was visualized as a pulsating bright red spike running in the midst of the heart wall from underneath of the left atrium towards the apex. Procedural consistency was maintained by ligating the left coronary artery, with a 7-0 silk suture and an atraumatic needle, ∼ 1 mm below the tip of the left auricle. Occlusion was confirmed by the immediate pallor of the anterior wall of the LV, regional hypokinesia and enlargement of the LV. The pericardium was returned as close as possible to its pre-opening state. The chest cavity was closed and the muscles and skin closed layer by layer with 4-0 silk sutures. Following extubation, mice were allowed to recover in an incubator set at 30 °C until they were fully ambulatory. The duration of the entire procedure was ∼ 15–20 min. Two-dimensional echocardiography Two-dimensional echocardiography (HDI 5000cv, Philips Ultrasound) was performed by a blinded investigator on sedated (1–1.5% isoflurane) mice using a high-frequency linear transducer (CL 15-7). Short-axis M-mode and two-dimensional images and loops of the LV at the mid-papillary muscle level were digitally acquired, stored and analyzed off-line. End diastolic posterior wall thickness and LV end diastolic diameter (LVEDD) were determined from frames taken at maximum cavity size. Dimensions of LV systolic diameter (LVESD) were recorded during maximum anterior motion of the posterior wall. Final values represent the average measurement of three consecutive cardiac cycles. Fractional shortening was defined as ((LVEDD−LVESD)/LVEDD) and LV ejection fraction was calculated from ((LVEDD 3 −LVESD 3 )/LVEDD 3 )×100. Haemodynamic measurements Closed-chest haemodynamic assessments were performed on anesthetized (1–1.5% isoflurane) mice. Mice were intubated and mechanically ventilated (133 cycles per min) with 100% oxygen. The LV was accessed with a 1.4F miniaturized impedance/micromanometer catheter (Millar Instruments) through the right carotid artery. The inferior vena cava was isolated immediately below the diaphragm for transient occlusion by applying gentle pressure with a cotton swab. LV pressure–volume relationships, acquired at a sampling rate of 1 kHz during steady state and transient occlusion of the inferior vena cava, were stored for off-line analysis. Calibration of volume signals from the conductance catheter was achieved by administration of 10% saline into the right jugular vein followed by calculation of the slope. External cuvette calibrations were also routinely performed to convert relative volume units to absolute volume measurements (in μl). Following study completion, the hearts were harvested and weighed before undergoing gross anatomical examinations. Determination of area at risk Evans blue (1.0%; Sigma) was injected retrograde through the abdominal aorta to delineate the non-ischaemic tissue before the heart was excised, washed with PBS and sliced into four transverse sections. Slices were stained for 20 min at 37 °C with 1.0 ml of 1.5% 2,3,5-triphenyltetrazolium chloride (Sigma) to determine the infarct area. Sections were photographed and the area at risk quantified with the aid of the NIH ImageJ software. Histology Histological studies were performed on hearts that were fixed in situ and stored in 3.7% paraformaldehyde or on hearts that were frozen in OCT and cryosectioned (5 μm). For gross histological examinations, sections (5–8 μm) were stained with haematoxylin and eosin. Infarct size was calculated as the ratio of total infarct to total endocardial circumference times 100. TUNEL staining was performed on deparaffinized sections either by routine DAB staining or with the Promega DeadEnd Fluorometric TUNEL kit and visualized by fluorescent confocal microscopy (Leica). The percentage of TUNEL-positive nuclei (per 1000) in each remote myocardial section was quantified and averaged from 5–7 randomly selected high-power (×400) fields. Other sections were examined via routine immunohistochemical methods using antibodies directed against BRCA1 (1:400; Santa Cruz), γH2A.X (1:100; Millipore), RAD51 (1:100; Millipore) and total caspase-3 (1:200; Cell Signaling). RNA measurements Total whole heart RNA was extracted with trizol reagent (Invitrogen) and reverse transcribed with the Quantitect Reverse Transcription Kit (Qiagen). Real-time reactions were carried out with a SYBR Green master mix on the PRISM 7900HT system (both Applied Biosystems) using the following primers: BRCA1 Forward-5′-ATCTGCCGTCCAAATTCAAG-3′ Reverse-5′-TTCCAAACAGATCGGACACTC-3′ Brain natriuretic peptide Forward-5′-ACAAGATAGACCGGATCGGA-3′ Reverse-5′-ACCCAGGCAGAGTCAGAAAC-3′ GAPDH Forward-5′-TGGATGCAGGGATGATGTTCT-3′ Reverse-5′-TGCACCACCAACTGCTTAGCC-3′ Western blotting Total protein, extracted with ice-cold RIPA buffer (Sigma) containing a protease inhibitor cocktail (Roche), was quantified with the Bio-Rad Protein Assay Reagent. Protein samples (50 μg) were separated by SDS-polyacrylamide gel electrophoresis, transferred to nitrocellulose membranes and probed with antibodies from Genway (BRCA1 (6B4), 1:750), Cell Signalling (p53; Bax; cleaved caspase-3; all at a 1:1000 dilution) or Millipore (Bcl-2, 1:1000; γH2A.X, 1:1000; GADPH, 1:4000; α-actin, 1:10,000). Following incubation with the appropriate horseradish peroxidase-associated secondary antibodies (Santa Cruz), signals were visualized with an enhanced chemiluminescence detection system (Amersham Bioscience) and quantified by densitometry. Human samples Approval was received from the Research Ethics Boards of St Michael's Hospital and the Hospital for Sick Children. Participation was voluntary and informed consent was obtained in all cases. Atrial samples were obtained from patients undergoing cardiac surgery with CP and CPB for coronary artery bypass graft surgery [30] . Pre-CP/CPB right atrial appendages were isolated using a double purse-string suture method during the placement of the venous cannula. Post-CP/CPB samples were collected after weaning from bypass and a brief period of reperfusion (5–15 min). Samples were flash frozen and processed for western blot and immunohistochemistry studies. Ventricular sections from sites distal to major coronary obstruction (patients undergoing coronary artery bypass graft surgery; ischaemic) and from sites with no clinical symptoms of ischaemia (patients undergoing valve replacement; non-ischaemic) were snap frozen and processed for immunohistochemical work. We ensured that the samples obtained for the ischaemic group were from areas that were chronically ischaemic yet viable, and not infarcted. They were from areas of the myocardium with planned revascularization. Semi-quantitative analysis to determine the extent of DAB staining in each section was performed with the ImageJ software ( http://rsb.info.nih.gov/ij/ ). Measurements were averaged to obtain a single value for each patient and in turn data from the patients in each group were averaged to obtain a single value for statistical analysis. Primary human fibroblast-conditioned media (HFCM) cultures were prepared from structurally normal hearts after elective pregnancy termination (gestational age, 15–20 weeks). Following enzymatic digestion with a 0.05% trypsin-collagenase solution (Life Technologies) at 37 °C, dissociated cells were concentrated from the supernatant and plated in 10% fetal bovine serum-supplemented Dulbecco's-modified Eagle's medium to allow for identification and removal of non-cardiomyocytes. This method yields cultures containing ∼ 80% β-myosin heavy chain-positive cardiac myocytes [31] . To simulate ischaemia, PBS-washed HFCM cultures were transferred to a pH 6.5 simulated solution containing 100 ml of deionized water, 0.8 g NaCl, 0.119 ml of N-2-hydroxyethylpiperazine-N-2-ethanesulfonic acid, 0.164 g 2-deoxyglucose, 0.89 ml KCl, 0.472 ml CaCl 2 , 0.238 ml of MgCl 2 and 0.135 ml of DL -lactic acid saturated in 100% N 2 for 1 h, followed by addition of 0.1 g of bovine serum albumin. After incubation for 24 h under 100% N 2 at 37 °C, HFCM cultures were processed for western blot analysis. Control HFCM cultures were maintained in fetal bovine serum-supplemented Dulbecco's-modified Eagle's medium at 37 °C in a standard CO 2 incubator. How to cite this article: Shukla, P. C. et al . BRCA1 is an essential regulator of heart function and survival following myocardial infarction. Nat. Commun. 2:593 doi: 10.1038/ncomms1601 (2011).